Ultrafast heating as a sufficient stimulus for magnetization reversal in a ferrimagnet The question of how, and how fast, magnetization can be reversed is a topic of great practical interest for the manipulation and storage of magnetic information. It is generally accepted that magnetization reversal should be driven by a stimulus represented by time-non-invariant vectors such as a magnetic field, spin-polarized electric current, or cross-product of two oscillating electric fields. However, until now it has been generally assumed that heating alone, not represented as a vector at all, cannot result in a deterministic reversal of magnetization, although it may assist this process. Here we show numerically and demonstrate experimentally a novel mechanism of deterministic magnetization reversal in a ferrimagnet driven by an ultrafast heating of the medium resulting from the absorption of a sub-picosecond laser pulse without the presence of a magnetic field. The fundamental limit of the speed of magnetization reversal is currently a topic of great interest, particularly for the magnetic storage industry [1] . It is generally accepted that magnetization reversal must be driven by a directional stimulus. Even the possibility to control the magnetic order parameter with the help of a time-invariant vector, for example, by an electric field, has recently become a subject of debate [2] , [3] . Previously, it has been assumed that heat can act only to assist magnetization reversal. Such thermally assisted magnetic recording in an external magnetic field is one of the most promising ways to enable recording of information at unprecedentedly high densities above 1Tb/inch 2 (ref. 4 ). This technology employs the effect of a laser-induced increase in the thermal energy of a magnetic medium in an external magnetic field. The necessity for the laser heating results from the large values of anisotropy required for thermal stability in recording media with small grain sizes, which are necessary to achieve the required signal to noise ratio at storage densities beyond 1Tb/inch 2 . Such large anisotropy values result in switching fields greater than the write fields available from current technology and the laser heating is used to produce a transient reduction in the anisotropy value to writable levels. Recent developments in near-field optics even allow laser-induced heating with extremely high precision below the diffraction limit [5] . The thermal assist brings the magnetic material into a state with an increased magnetic susceptibility, but the actual magnetization reversal and recording is driven by the simultaneously applied external magnetic field. In recent years, owing to an increased interest in ferrimagnetic materials, there have been a number of studies of ultrafast magnetic switching based on increasing the temperature of a ferrimagnetic material over its magnetic compensation point with the help of a short laser pulse [6] , [7] , [8] . These studies demonstrated a strongly increased magnetic susceptibility followed by thermally assisted magnetization reversal in an external magnetic field. Such an increased susceptibility could not be defined in terms of equilibrium thermodynamics. Very recently, it has been discovered that such a thermal-energy increase of a ferrimagnet over the compensation point brings the system into a strongly non-equilibrium, transient ferromagnetic-like state [9] . This raises the question of what is the actual magnetic susceptibility of this novel non-equilibrium state and what is the minimum external magnetic field required to trigger magnetization reversal? Aiming to answer these questions, we arrived at the counterintuitive and very intriguing conclusion that magnetization reversal could be achieved without any magnetic field, using an ultrafast thermal energy load alone. Intuitively, this conclusion seems to be contradicting since it is not clear how a thermal-energy increase, that is not a vector quantity, can result in a deterministic reversal of a vector. Nevertheless, if a novel mechanism of magnetic recording by ultrafast thermal energy load alone were possible, it would open up the possibility to combine Tb/inch [2] , densities with THz writing rates, while using much less power because it would not require the application of a magnetic field. To verify the feasibility of such a hypothetical magnetization reversal scenario, we performed atomistic scale modelling of laser-induced spin dynamics in a Heisenberg Gd–Fe ferrimagnet. The numerical results support the above conjecture. Specifically, it is demonstrated that magnetization can be reversed after the application of femtosecond laser pulses that increase the temperature of the thermal bath very rapidly in the absence of an applied field. The rapid transfer of thermal energy into the spin system leads to switching of the magnetization within a few picoseconds. Importantly for technological applications, we show, numerically and experimentally, that this type of switching can occur when starting at room temperature. The simulations show that such a switching process proceeds with such impetus that even an opposing 40 T field is not able to prevent the magnetization from reversing on a short timescale. This switching mechanism has been experimentally verified in isolated in-plane and out-of-plane microstructures of GdFeCo under the action of a sequence of linearly polarized laser pulses. A further set of experiments showing the importance of the heat generation is presented, whereby we show, using circularly polarized laser pulses that this switching occurs independently of polarization and initial state in thin films of GdFeCo. Atomistic modelling of sub-picosecond switching without a field In the atomistic model, we incorporate the rapid change in thermal energy of a system under the influence of a femtosecond laser pulse, and include the antiferromagnetic exchange interaction between the two magnetic sublattices. The atomistic spins are coupled to the temperature of the electron thermal bath [10] , [11] , the temporal evolution of which is calculated using the two temperature model [12] . The electronic thermal bath is coupled to that of the phonons, whereby thermal energy is removed from the electronic system on the picosecond timescale. The phonon thermal bath is also coupled to an external bath of constant temperature at 300 K that is above the compensation point of the simulated alloy. This thermal bath equilibrates the temperature back to its starting value on the nanosecond timescale. The action of a femtosecond laser pulse in the simulation results in a rapid change in the electronic temperature, to which we couple the spin system. 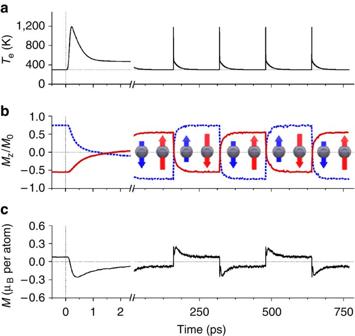Figure 1: Computed ultrafast thermally induced switching dynamics. (a) Evolution of the temperature of the electronic thermal bath during a sequence of 5 Gaussian pulses. (b) Computed time-resolved dynamics of the z-component of the magnetizations of Fe and Gd sublattices; Gd is represented by the solid red line and the Fe by the dashed blue line. The net magnetization is shown in (c). A spike in the temporal behaviour of the total magnetization during the excitation is due to different dynamics of the magnetizations of the Fe and Gd sublattices as reported in (ref.9). Figure 1a shows how the electronic temperature varies with time during the action of 5 successive Gaussian thermal pulses with a temporal width of 50fs each. We have simulated the collective response of the spins in the ferrimagnet Gd–Fe to an ultrafast linearly-polarized pulse. Figure 1b shows the z component of the magnetization for the individual Fe and Gd sublattices. Figure 1c shows the z component of the net magnetization. The results clearly show that the magnetic order parameter of the ferrimagnet is switched every time a pulse is applied to the system without the need for the application of a magnetic field. Figure 1: Computed ultrafast thermally induced switching dynamics. ( a ) Evolution of the temperature of the electronic thermal bath during a sequence of 5 Gaussian pulses. ( b ) Computed time-resolved dynamics of the z-component of the magnetizations of Fe and Gd sublattices; Gd is represented by the solid red line and the Fe by the dashed blue line. The net magnetization is shown in ( c ). A spike in the temporal behaviour of the total magnetization during the excitation is due to different dynamics of the magnetizations of the Fe and Gd sublattices as reported in (ref. 9 ). Full size image The timescale for this switching indicates that this phenomenon cannot be explained in terms of what is currently known for the timescale of the spin–orbit interaction and thus must be driven by the exchange interactions in the spin system. To this end we have also performed numerical calculations to gauge the strength of this reversal mechanism. 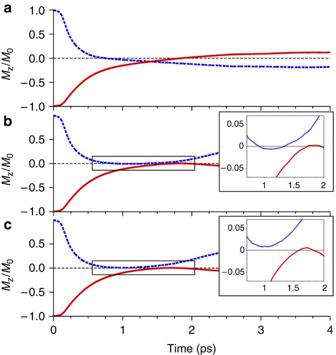Figure 2: Computed time-resolved dynamics of the z-component of the Fe and Gd sublattice from localized atomistic spin model. (a–c) Dynamics of the Fe (blue dashed lines) and Gd (red solid lines) sublattice with applied fields of 10, 40 and 50 T, respectively, to prevent reversal of the Fe sublattice. The system is initially in the anti-parallel ground state at 0 K and a Gaussian laser pulse is applied driving the system into a non-equilibrium state whereby the sublattices attempt to align against the exchange interaction and the applied field. Figure 2 shows the simulated time-resolved magnetization dynamics for the Fe and Gd sublattices while an opposing field was applied to prevent reversal of the Fe sublattice against the exchange interaction from the Gd sublattice. The critical strength of applied field was calculated to be dependent on the system properties and the intensity of the laser pulse. Figure 2a–c shows the magnetization dynamics of the individual sublattices in an opposing 10, 40 and 50 T applied field, respectively. As Figure 2b shows, a field of 40 T is still insufficient to prevent the reversal. Figure 2: Computed time-resolved dynamics of the z-component of the Fe and Gd sublattice from localized atomistic spin model. ( a – c ) Dynamics of the Fe (blue dashed lines) and Gd (red solid lines) sublattice with applied fields of 10, 40 and 50 T, respectively, to prevent reversal of the Fe sublattice. The system is initially in the anti-parallel ground state at 0 K and a Gaussian laser pulse is applied driving the system into a non-equilibrium state whereby the sublattices attempt to align against the exchange interaction and the applied field. Full size image Experimental verification in thin films of GdFeCo We have experimentally verified this switching mechanism by studying the response of ferrimagnetic Gd 24 Fe 66.5 Co 9.5 to the action of 100 fs laser pulses, with an experimental setup similar to that described elsewhere [13] . The small amount of Co (9.5%) is added to control the perpendicular anisotropy of the film. In the experiments, the alloy was excited with several 100 fs laser pulses, and the final magnetic state was recorded using a magneto-optical microscope, which is sensitive to the out-of-plane orientation of the FeCo sublattice via the magneto-optical Faraday effect. Here we detect the direction of the FeCo magnetization in the steady state, long after the excitation event, so that the Gd and FeCo magnetizations are anti-parallel. 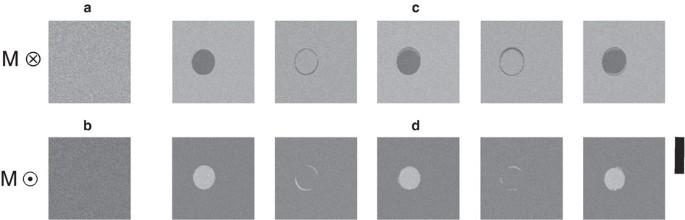Figure 3: The magneto-optical images of a Gd24Fe66.5Co9.5continuous film obtained after the action of a sequence of N 100 fs laser pulses. (a) and (b) Initial homogeneously magnetized state of the film with magnetizations 'up' and 'down' as represented by the circled dot and cross respectively. The light grey region represents magnetization pointing 'down' and the darker grey 'up'. (c) and (d) The film after an excitation withN(N=1, 2...5) pulses with a fluence of 2.30 mJ cm−2. Each laser pulse excites the same circular region of the film and reverses the magnetization within it. The scale bar on the right corresponds to 20 μm. Figure 3 shows the result of the action of a sequence of laser pulses on the continuous film of Gd 24 Fe 66.5 Co 9.5 , initially in a single domain state with magnetization perpendicular to the sample surface. In this figure, light grey areas correspond to domains magnetized 'down' ( Fig. 3a ), whereas dark grey areas correspond to the domains magnetized 'up' ( Fig. 3b ). Looking at the Fig. 3c , after excitation of the light-grey region with the very first pulse, one can see the formation of a dark-grey domain. The second pulse then reverses the magnetization of the excited area forming a light grey domain. Every such pulse thereafter triggers this reversal. The opposite is seen in Figure 3d , beginning in the opposite state. The experimental observations are in excellent agreement with the switching predicted by the atomistic simulations, where every pulsed excitation should trigger the magnetization reversal. Figure 3: The magneto-optical images of a Gd 24 Fe 66.5 Co 9.5 continuous film obtained after the action of a sequence of N 100 fs laser pulses. ( a ) and ( b ) Initial homogeneously magnetized state of the film with magnetizations 'up' and 'down' as represented by the circled dot and cross respectively. The light grey region represents magnetization pointing 'down' and the darker grey 'up'. ( c ) and ( d ) The film after an excitation with N ( N =1, 2...5) pulses with a fluence of 2.30 mJ cm −2 . Each laser pulse excites the same circular region of the film and reverses the magnetization within it. The scale bar on the right corresponds to 20 μm. Full size image It is important to note that the observed sequence of switching occurs independently of the polarization of the laser pulses, as shown in Supplementary Figure S1a,b . The observed magnetization switching that occurs independently of the initial state of the magnetization and light polarization eliminates an explanation via the involvement of the time-non-invariant and light-induced effective field H IFE ~ E×E * , which results from the inverse Faraday effect [14] . We have found that this laser-induced switching is observed for pump fluences just above the window of fluences required for all-optical helicity-dependent switching reported in ref. 13 , where control of the magnetization orientation requires the presence of a light-induced effective field H IFE . In fact, in the present experiment, the all-optical helicity-dependent reversal is responsible for the thin rim with switched magnetization observed after each even laser pulse ( Fig. 3 ; Supplementary Figs S1a,b and S2 ). Therefore, our experimental results demonstrate that excitation of ferrimagnetic GdFeCo with a sufficient intensity always results in magnetization reversal, independent of the polarization of the laser pulse. The experiments were carried out at room temperature (300 K), while the magnetization compensation temperature for the given alloy is 280 K. This excludes an explanation of the reversal as a result of a temperature increase through the compensation point [8] . This observation is supported by the numerical model ( Supplementary Fig. S3 ) and discussed further in the Supplementary Methods section ( Supplementary Fig. S2 ). Experimental verification in lithographically patterned media One may argue that this helicity-independent, all optical magnetization reversal is not necessarily driven by heating alone, as predicted by the atomistic simulations, but rather a switching driven by the interplay of heat with stray fields and/or domain walls created in the region surrounding the illuminated area [15] . To exclude the possibility of such artefacts, arrays of 2μm diameter disks of Gd 25 Fe 65.6 Co 9.4 were fabricated. The size was chosen so that the structures are much smaller than the laser spot size of about 30×100 μm (full-width at half-maximum) and so that several structures can be investigated simultaneously within the same field of view of the microscope and excited by the very same laser pulse. The distance between the structures is as large as their diameter, thereby reducing dipolar interactions between them to a negligible degree. No correlations between the magnetization directions of neighbouring structures were observed. The magnetization direction in these microstructures was measured with a photoemission electron microscope (PEEM) employing the X-ray magnetic circular dichroism (XMCD) effect. First, structures with an out-of-plane anisotropy, similar to the continuous film above, were studied and XMCD images recorded at the Fe L 3 edge (708 eV) are shown in Fig. 4a . Displayed are two microstructures, one with dark grey and one with a light grey contrast, which correspond to magnetizations pointing in opposite directions, that is, up and down, respectively, out of the sample plane. Starting from the initial state ( Fig. 4a ), we applied a series of linearly polarized femtosecond laser pulses. After the first single pulse, the contrast is simultaneously reversed in both structures, meaning that the magnetization has switched relative to the initial state. This magnetization reversal occurs after every subsequent single laser pulse. With the same laser pulse the magnetization in one structure is switched from up to down while in the other structure it is switched from down to up. In the simulations, the reversal occurs regardless of the strength of the uniaxial anisotropy (for anisotropy fields within reasonable limits) and regardless of whether the anisotropy is in-plane or out-of-plane. We have, therefore, also investigated in-plane magnetized microstructures. The XMCD images are shown in Fig. 4b with the bright and dark contrast corresponding to opposite in-plane magnetization directions. The contrast in both structures reverses after every laser pulse, meaning that the magnetization switches every time the micro-structures are excited with a single laser pulse. Again, structures with opposite magnetization directions reverse simultaneously. We point out that the structures are in an as-grown state and that they are not coupled to each other by stray fields. We do observe the switching also for neighbouring structures pointing in the same direction regardless of whether the sample was demagnetized or magnetized before the measurement. All these experiments thus demonstrate that the ultrafast thermal energy increase created by a laser pulse of any polarization induces a deterministic switching of the magnetization, without the need for any other external stimulus. 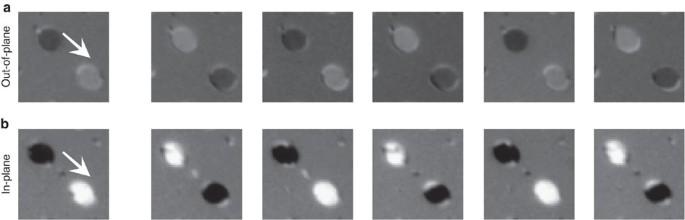Figure 4: XMCD images at Fe L3edge of 2 μm wide Gd25Fe65.6Co9.4structures. (a) Images of microstructures with out-of-plane anisotropy, magnetized perpendicular to the sample plane. The first image in (a) shows the initial state of the microstructures where the magnetization of the darker structure points down while the magnetization of the brighter one points up. The next image is taken after excitation with a single linearly polarized laser pulse and shows that the magnetizations of both elements are reversed. This reversal occurs after every laser pulse, as can be seen in the subsequent images in (a). (b) Images of microstructures with in-plane anisotropy. The bright and dark areas correspond to magnetization directions in the plane of the sample pointing parallel or anti-parallel to the X-ray direction. The subsequent images are taken after each excitation with a single linearly polarized laser pulse demonstrating the reversal of the magnetization. The X-ray direction is indicated by an arrow and the structures have a size of 2 micrometers. Figure 4: XMCD images at Fe L 3 edge of 2 μm wide Gd 25 Fe 65.6 Co 9.4 structures. ( a ) Images of microstructures with out-of-plane anisotropy, magnetized perpendicular to the sample plane. The first image in ( a ) shows the initial state of the microstructures where the magnetization of the darker structure points down while the magnetization of the brighter one points up. The next image is taken after excitation with a single linearly polarized laser pulse and shows that the magnetizations of both elements are reversed. This reversal occurs after every laser pulse, as can be seen in the subsequent images in ( a ). ( b ) Images of microstructures with in-plane anisotropy. The bright and dark areas correspond to magnetization directions in the plane of the sample pointing parallel or anti-parallel to the X-ray direction. The subsequent images are taken after each excitation with a single linearly polarized laser pulse demonstrating the reversal of the magnetization. The X-ray direction is indicated by an arrow and the structures have a size of 2 micrometers. Full size image The scenario of the reversal can be understood as follows. An ultrashort laser pulse increases the thermal energy of the electronic system in metallic GdFeCo, creating a thermal bath for spins with a temperature much higher than the Curie point. The rapid increase in thermal energy of the system leads to a very fast energy transfer into the spin system. This results in the Fe and Gd sublattices demagnetizing on very different timescales mainly because of the differing magnetic moments. In the background of these processes, the temperature of the electronic system rapidly decreases as a result of electron–phonon interaction, and, after less than 1 ps, the temperature is below the Curie temperature. After this initial sharp increase of the temperature of the electronic heat bath, the magnetization of the sublattices is still changing due to exchange relaxation [16] . The non-equivalence of the sublattices combined with the exchange relaxation means that the Fe reaches zero magnetization before that of Gd, eventually leading to the onset of the ferromagnetic-like state where the two sublattices align parallel, observed in ref. 9 . The magnetization of the Fe sublattice is then increasing while the Gd is decreasing because of the exchange relaxation. As the antiferromagnetic exchange from the Gd is weaker than the ferromagnetic ordering in Fe, the Gd reverses at a longer timescale due to the inter-sublattice exchange. The exchange-driven relaxation of the system from the strongly non-equilibrium state to a partial equilibrium will stimulate the reversal of the total magnetization of the material. Following this, the system evolves from this partial equilibrium to the complete equilibrium during the timescale of interactions of relativistic origin. The non-equivalence of the sublattices and their corresponding different demagnetization times are essential for the process presented here. To demonstrate the importance of the sublattice non-equivalence at this stage of the reversal process, we performed numerical simulations making the local moments on each site equal. No reversal occurs in this case ( Supplementary Fig. S4 ). The novel magnetization reversal mechanism that we have presented is expected to be typical for magnets with at least two non-equivalent magnetic sublattices coupled by an antiferromagnetic exchange interaction. Even though the two sublattices are exchange coupled, they still demagnetize at different rates as in their pure ferromagnetic form [17] , [18] . This non-equivalence of the sublattices is essential for the reversal, requiring different rates of demagnetization in each sublattice. The mechanism does not require the presence of any other stimulus and occurs each time a laser pulse excites the magnetic sublattices of a ferrimagnet. This mechanism of magnetization reversal is demonstrated experimentally with starting temperatures above and below the magnetization compensation temperature in GdFeCo continuous films and also for microstructures with in-plane and out-of-plane magnetic anisotropy. Also relevant for technological applications, we have shown numerically and experimentally that switching can occur when the sample is at room temperature before laser excitation. One can therefore imagine a magnetic recording system with magnetic bits recorded using a thermal pulse alone, removing the necessity for the inductive write head, which presently forms a serious limitation on recording densities. Because the simulations were carried out on ~30 nm 3 systems, we see no reason why this material or others like it could not be used for recording media on the nanometre scale, the requirement for high-density recording. The results presented here may allow both higher recording densities as well as increased data rates, as the recording of a bit could be achieved on a timescale of picoseconds rather than the current nanoseconds. Atomistic modelling The localized atomistic model of GdFe is parameterized on experimental observations, with the essential parameters fitted accordingly [19] . It is seen experimentally that Gd and Fe form two sublattices that are aligned anti-parallel in the ground state. This means that we have antiferromagnetic exchange between the Fe and Gd and that the intra-sublattice exchange parameters are ferromagnetic. The energetics of any spin in the system, i are described by the Hamiltonian. Where J ij is the exchange integral between spins, i and j ( i,j are lattice sites) giving rise to magnetic order on the system; S i is the normalized spin vector | S i |=1; d , is the uniaxial anisotropy constant; N is the number of nearest neighbours. We model the magnetization dynamics of the system through the use of the Landau–Lifshitz–Gilbert equation [20] with Langevin dynamics, given by; Here λ i and γ i are the microscopic thermal bath coupling parameter and the gyromagnetic ratio, respectively; μ i is the magnetic moment of the site, i. The effective field H i , is then given by: Here ζ i ( t ) is a stochastic term, which describes the coupling of the spin system to the external thermal bath. The thermal fluctuations are included as a white noise term, uncorrelated in time and space, which is added into the effective field. The stochastic integrals are interpreted as Stratonovich integrals [21] . The moments of the stochastic process are defined through fluctuation dissipation theory as: Here a , b are Cartesian components; T is the temperature of the thermal bath to which the spins are coupled. The coupling of the spins to the thermal bath ( λ i ) is a parameter that attempts to describe all of the energy and momentum transfer channels into the spin system, for example, from the conduction electrons. To model the alloys amorphous character, we randomly pick Fe sites and replace them with Gd impurities [19] . The composition for all of the numerical simulations, presented in this manuscript, is Fe 76 Gd 24 . For each of the Fe and Gd spins, we write a Landau–Lifshitz–Gilbert equation (~10 6 equations in total) and solve it using the Heun numerical integration scheme. The exchange constants, anisotropy constants and the gyromagnetic ratio of the sublattices for the modelled Heisenberg Gd–Fe magnet were taken similar to those used in ref. 9 . They were J Fe − Fe =2.835×10 −21 J, J Gd − Gd =1.26×10 −21 J (corresponding to the Curie temperature of bulk Gd) and J Fe − Gd =−1.09×10 −21 J. The gyromagnetic ratios of the Gd and Fe sublattices were set to γ Fe =1.05 γ and γ Gd = γ , with γ=1.76×10 11 T −1 S −1 . Following ref. 10 , we couple the spin system to the electron temperature that is calculated using the so-called two-temperature model [12] . For simplicity, the model assumes the same electron temperature and the same damping constants for Gd and Fe (λ Fe = λ Gd =0.01). In the atomistic model, we have ignored the role of the Cobalt as XMCD measurements show that the Fe and Co are coupled ferromagnetically. Experimentally Cobalt is added to improve the Faraday signal. Field required to prevent reversal We performed numerical calculations, whereby, throughout this particular calculation, a field is applied to prevent the formation of the transient ferromagnetic-like state reported in this type of material [9] . To achieve this, we augmented equation (1) with the Zeeman term, μ i B where B is the applied field. In these simulations, starting at a temperature of 0 K, the electronic temperature is increased through the magnetization compensation temperature T M =250 K up to a peak before dropping down to the final temperature at around 350 K. At this temperature, the Fe sublattice has the largest magnetization. To prevent its reorientation, we applied a magnetic field in the direction initially aligned with the Fe sublattice. The pulse is assumed to be Gaussian in time and space in the numerical simulations. Starting from 0 K, the Gaussian thermal pulse is coupled to the electronic temperature through the two-temperature model [12] . The field strength, required to prevent reversal of the Fe sublattice, is dependent on the measurement time window, as the system will start to precess to align with the field. As a limiting case, we can consider the timescale of the order of 1 ns, which is a characteristic time for the precessional reversal. At this timescale, the field required to prevent reversal is equal to the intrinsic anisotropy of the system. 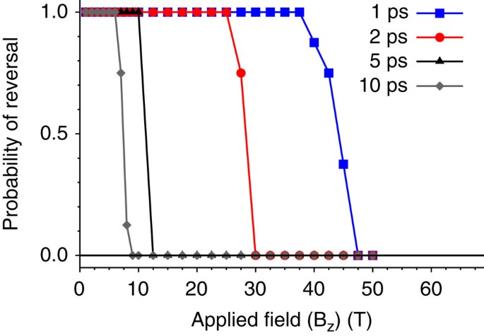Figure 5: Numerical calculations showing the magnetic field required to prevent reversal of the Fe sublattice. The required field depends on the time at which the magnetization is measured as precessional reversal starts to push the magnetization back into alignment with the applied field. Each point is averaged over 100 runs, each with a different seed for the random number generator, for the placing of the Fe and Gd moments and for the thermal term. Each run begins at 0 K and with the electronic temperature increasing rapidly before dropping below the Curie temperature. Figure 5 shows the field required to prevent reversal when the magnetization is taken at 1, 2, 5 and 10ps. It can be seen that a field of around 40 Tesla is required to prevent the Fe magnetization from reversing into the Gd direction (that is, the transient ferromagnetic-like state) at a delay of 1 ps. Depending on the time at which the measurement is made, the field required to prevent reversal changes. Numerical simulations also show that the field required to prevent reversal depends on the input parameters, for example, the coupling parameter ( λ i ), as described by equation (4). Figure 5: Numerical calculations showing the magnetic field required to prevent reversal of the Fe sublattice. The required field depends on the time at which the magnetization is measured as precessional reversal starts to push the magnetization back into alignment with the applied field. Each point is averaged over 100 runs, each with a different seed for the random number generator, for the placing of the Fe and Gd moments and for the thermal term. Each run begins at 0 K and with the electronic temperature increasing rapidly before dropping below the Curie temperature. Full size image Sample preparation of microstructures The structures are produced via a lift-off technique [22] . A polymethylmethacrylate resist is first patterned with an electron beam writer on a glass/Ti(2 nm)/Pt(8 nm) substrate. This pattern is then transferred via lift-off after deposition by magnetron sputtering of the magnetic multilayer AlTi(10 nm)/Si 3 N 4 (5 nm)/Gd 24 Fe 66.6 Co 9.4 (20 nm)/Si 3 N 4 (3 nm), resulting in isolated magnetic structures [23] . Unstructured areas of several 100 μm, quasi-continuous films, and arrays of squares and disks down to 1 μm were fabricated onto the same sample. In the manuscript, we focus only on the 2 μm disks, but the reversal of the magnetization direction, after applying a single laser pulse, was observed in the continuous film part as well as in the structures down to 1 μm. PEEM measurements The magnetization direction in these microstructures was measured with a PEEM from Elmitec GmbH at the SIM beamline [24] of the Swiss Light Source at the Paul Scherrer Institut (PSI) employing the XMCD effect. An XMCD image is obtained by taking the ratio of two total electron yield images measured with opposite helicities at resonant energies, and the resulting contrast is proportional to the scalar product of the local magnetization and the incoming X-ray wave vectors [25] , that is, the more parallel the magnetization is to the X-ray wave vector, the brighter the contrast. As the incident angle of the X-rays is 16°, with respect to the surface, a magnetization in the plane of the sample surface has a stronger contrast compared with a magnetization pointing out of the surface plane, and an azimuthal-dependent XMCD study enables the determination of a three-dimensional (3D) map of the local magnetization [26] . Such a study allows us to confirm whether the magnetization is in-plane or out-of-plane. The elemental selectivity of XMCD allows the determination of the magnetization direction of the two ferromagnetic sublattices. For the 3d metal sublattice, the X-rays are tuned to the Fe L 3 edge (708 eV) and for the 4f sublattice to the Gd M 5 edge (1190 eV). These measurements confirmed the antiparallel coupling between the Fe and Gd sublattices. The spatial resolution in the XMCD images is about 100 nm. The structures in Figure 4 are not exactly round because of a small misalignment of the imaging stigmators and some imperfections during the sample production. The contrast at the outer rim of the structures indicates small areas with a different magnetization direction compared with the centre part. For the laser excitation, an XL-500 oscillator from FEMTOLASERS GmbH, producing 50 fs laser pulses, at 5.2 MHz repetition rate, was used. The laser power required for switching the magnetization was set using a half wave plate in combination with a polarizer. Single pulses are selected by a pulse-picker and the laser impinges onto the sample with 16° grazing incidence. How to cite this article: Ostler, T.A. et al . Ultrafast heating as a sufficient stimulus for magnetization reversal in a ferrimagnet. Nat. Commun. 3:666 doi: 10.1038/ncomms1666 (2012).